Reply to ‘Forward models of repetition suppression depend critically on assumptions of noise and granularity’ 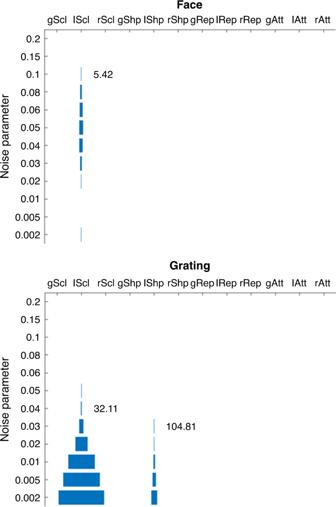Fig. 1: The effect of noise on model fits. This figure shows which models (x-axis) could fit the data from each experiment as a function of the noise parameter (y-axis) after an exhaustive grid search of values for five parameters (σNoise,N,a,bandσ; see text). The width of the horizontal bars reflects the number of unique sets of parameter values that could fit the data patterns for each model (for a given noise level). The number to the right of bars shows the lowest signal-to-noise ratio (SNR) achievable (at the location of the corresponding noise parameter value). Note that the SNR is related to the noise parameter, but also depends on the other model parameters, which affect the signal, so does not necessarily occur at the lowest noise parameter value. The range of parameter values explored wereN= [4 8 16 32],a= [0.1 0.2 0.3 0.4 0.5 0.6 0.7 0.8 0.9],b= [0.1 0.3 0.5 0.7 0.9 1.1 1.3] andσ= [0.1 0.3 0.5 0.7 0.9 2 4 6 8 10] (unique noise parameter values shown ony-axis). The important point is that only the local scaling model could fit the face data (up to SNRs of 5.42), and while local sharpening could also fit the grating data, as Ramirez and Merriam noted, it required a higher SNR (104.81) and did so with fewer sets of parameter values. Acronyms on thex-axis stand for (from left to right) the following models: global scaling, local scaling, remote scaling, global sharpening, local sharpening, remote sharpening, global repulsion, local repulsion, remote repulsion, global attraction, local attraction and remote attraction. Further information on research design is available in the Nature Research Reporting Summary linked to this article.